Postnatal muscle modification by myogenic factors modulates neuropathology and survival in an ALS mouse model MyoD and myogenin are myogenic transcription factors preferentially expressed in adult fast and slow muscles, respectively. Amyotrophic lateral sclerosis (ALS) is a neurodegenerative disorder in which motor neuron loss is accompanied by muscle denervation and paralysis. Studies suggest that muscle phenotype may influence ALS disease progression. Here we demonstrate that myogenin gene transfer into muscle supports spinal cord motor neuron survival and muscle endplate innervation in the G93A SOD1 fALS mice. On the other hand, MyoD gene transfer decreases survival and enhances motor neuron degeneration and muscle denervation. Although an increase in motor neuron count is associated with increased succinic dehydrogenase staining in the muscle, muscle overexpression of PGC-1α does not improve survival or motor function. Our study suggests that postnatal muscle modification influences disease progression and demonstrates that the muscle expression of myogenic and metabolic regulators differentially impacts neuropathology associated with disease progression in the G93A SOD1 fALS mouse model. Amyotrophic lateral sclerosis (ALS) is a progressive neurodegenerative disorder characterized by the loss of upper and lower motor neurons. Motor neuron losses are accompanied by muscle weakness and paralysis. A number of clinical studies have reported increased vulnerability of fast-fatiguable motor units in ALS patients [1] , [2] . Studies of muscle fibre phenotype [3] and motor units [4] in transgenic mice overexpressing mutant G93A human SOD1 (G93A mice) indicate that fast muscles are preferentially affected. These findings suggest that muscle phenotype may have an influence on ALS neuropathology. However, the role of muscle in ALS pathogenesis remains ambiguous. Although muscle specific expression of mutant SOD1 results in motor neuron loss and muscle denervation [5] , [6] , Cre-mediated partial knockdown of mutant SOD1 in the muscle did not have an impact on the disease progression [7] . Still, early changes in muscle biochemistry and the effectiveness of muscle-specific expression of either GDNF or IGF-1 in mediating motor neuron rescue and delay in the disease progression in these mice suggest a potentially important and influential role of the muscle on the disease progression [8] . MyoD and myogenin are muscle regulatory factors involved in muscle development and differentiation [9] , [10] . In adult muscle, MyoD is mainly expressed in adult fast muscle fibres [11] , [12] , [13] and regulates fast muscle development [12] . On the other hand, myogenin is predominantly expressed in slow muscle fibres [11] , [13] and its expression increases oxidative metabolism in muscle [14] , [15] . Another factor that has been shown to be a modulator of muscle phenotype is peroxisome proliferator-activated receptor gamma coactivator-1α (PGC-1α). PGC-1α is a potent metabolic regulator of muscle and its expression enhances slow oxidative muscle phenotype [16] . In this study we examined whether postnatal modification of muscle phenotype can modify disease progression in the G93A SOD1 fALS mouse model; adult muscle is highly plastic and can be phenotypically remodelled by intrinsic and extrinsic cues [17] , [18] . We show that postnatal modulation of muscle phenotype as a consequence of exogenous expression of MyoD or myogenin in hindlimb muscles of adult G93A mice modulates motor neuron degeneration, muscle denervation and survival. On the other hand, muscle overexpression of PGC-1α does not improve survival or motor function in these mice. Our results demonstrate that disease progression in a fALS mouse model can be either improved or worsened through postnatal muscle modification, and also demonstrate that myogenic and metabolic factors in the muscle differentially influence the clinical outcome in the G93A mice. MyoD gene transfer accelerates disease progression We exogenously expressed MyoD in the hindlimb muscles of adult male G93A mice using adenovirus expressing human MyoD (ad-MyoD) and investigated the effect on motor behaviour. Gene transduction efficiency following virus-mediated gene transfer into muscle was determined using adenovirus expressing LacZ. Two weeks following injection, ~16% of the muscle fibres were X-gal-positive in the gastrocnemius muscle ( Fig. 1a ). The number of muscle fibres positive for LacZ stain decreased over time, demonstrating the transient nature of resulting LacZ gene expression ( Fig. 1a ). Examination of the lumbar portion of spinal cord did not show any X-gal staining, suggesting that the virus injected into the hindlimb muscles is not retrogradely taken up by motor neurons in our study ( Fig. 1b ). 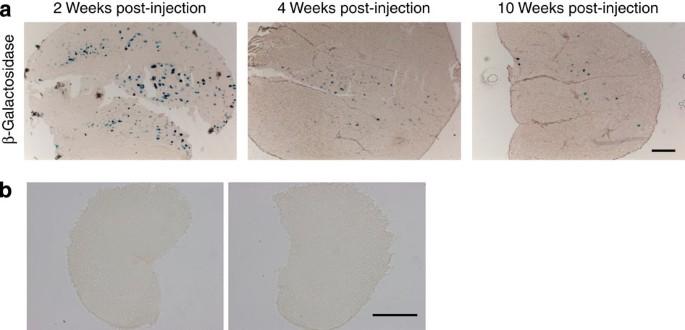Figure 1: Efficiency of adenovirus-mediated gene transfer into adult muscle was determined in the gastrocnemius muscle using β-galactosidase construct. (a) A single injection resulted in widely distributed gene expression 2 weeks post injection. Stereological counting showed that ~16% of the muscle fibres were visibly stained for β-galactosidase (blue). The gene expression level declined over time showing the transient nature of the β-galactosidase gene expression. (b) Examination of the lumbar portion of the spinal cord at 2 weeks post injection did not show any X-gal staining, demonstrating that virus is not retrogradely transported into motor neurons following virus injection. Scale bar represent 500 μm. Figure 1: Efficiency of adenovirus-mediated gene transfer into adult muscle was determined in the gastrocnemius muscle using β-galactosidase construct. ( a ) A single injection resulted in widely distributed gene expression 2 weeks post injection. Stereological counting showed that ~16% of the muscle fibres were visibly stained for β-galactosidase (blue). The gene expression level declined over time showing the transient nature of the β-galactosidase gene expression. ( b ) Examination of the lumbar portion of the spinal cord at 2 weeks post injection did not show any X-gal staining, demonstrating that virus is not retrogradely transported into motor neurons following virus injection. Scale bar represent 500 μm. Full size image In our first set of experiments, mice were injected with either ad-MyoD or ad-GFP. Expression of human MyoD in the muscle following adenoviral construct injection was confirmed using qPCR ( Fig. 2a ; t- test, P <0.00001, n =4 samples per group). The behavioural effect of MyoD overexpression in hindlimb muscles of G93A mice was determined through a weekly assessment of rotarod performance and weight measures starting at 56 days of age. A comparison of the ad-MyoD injection group ( n =9) with the ad-GFP injection group ( n =9) showed a statistically significant difference in the temporal profile of latency-to-fall on rotarod ( Fig. 2b , two-way ANOVA, F (1,140)=23.33; P <0.0001; n =9 mice per group). Bonferroni post-test showed statistically significant difference in the rotarod performance between the two groups at 91 days ( P <0.05), 98 days ( P <0.05) and 105 days ( P <0.001) of age. Weight loss parallelled the temporal pattern of rotarod performance. Ad-MyoD-injected mice displayed faster weight loss than ad-GFP-injected mice ( Fig. 2c , two-way ANOVA, F (1,140)=3.390; P =0.0014; n =9 mice per group). The differences were statistically significant starting at 105 days (Bonferroni post-test; 105 days, P <0.05; 112 days, P <0.01; n =9 mice per group). Concomitantly, the survival rate was significantly reduced in ad-MyoD-treated mice ( Fig. 2d , Kaplan–Meier curve, log ranking, P =0.0018; n =9 mice per group) and on average reached the endpoint 11% faster (110.56 days versus 124.57 days, unpaired two-tailed t -test, P =0.003; n =9 mice per group). Therefore, postnatal expression of MyoD in hindlimb muscles accelerates motor abnormalities as well as weight loss in G93A mice and decreases survival. 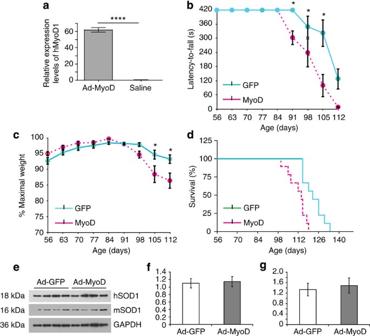Figure 2: MyoD gene transfer into Adult G93A hindlimb muscle accelerates rotarod deficit and weight loss. (a) Expression of human MyoD1 in the muscle following adenoviral construct injection was confirmed using quantitative real-time PCR (n=4 per group,t-test, ****P<0.00001). (b) Rotarod latency-to-fall is decreased at 20 r.p.m. for Ad-MyoD-injected mice starting at 91 days of age compared with ad-GFP-injected mice (two-way ANOVA,F(1,140)=23.33,P<0.0001; *P≤0.05, Bonferronipost hoctest,n=9 mice per group). (c) Weight-loss in ad-MyoD-injected mice was also greater starting at 98 days of age compared with ad-GFP-injected group (two-way ANOVA,F(8,140)=3.390,P=0.0014; *P≤0.05, Bonferroni test,n=9 mice per group). (d) Survival is reduced in ad-MyoD-injected mice (Kaplan–Meier analysis, log-rank,P=0.0018). ad-MyoD (dashed line); ad-GFP (solid line);n=9 mice per group. (e) Western blotting shows that neither the mutant SOD1 (f, hSOD1) nor the mouse SOD1 (g, mSOD1) is altered following MyoD gene transfer (n=4 samples per group). Data are presented as mean±s.e.m. Figure 2: MyoD gene transfer into Adult G93A hindlimb muscle accelerates rotarod deficit and weight loss. ( a ) Expression of human MyoD1 in the muscle following adenoviral construct injection was confirmed using quantitative real-time PCR ( n =4 per group, t -test, **** P <0.00001). ( b ) Rotarod latency-to-fall is decreased at 20 r.p.m. for Ad-MyoD-injected mice starting at 91 days of age compared with ad-GFP-injected mice (two-way ANOVA, F (1,140)=23.33, P <0.0001; * P ≤0.05, Bonferroni post hoc test, n =9 mice per group). ( c ) Weight-loss in ad-MyoD-injected mice was also greater starting at 98 days of age compared with ad-GFP-injected group (two-way ANOVA, F (8,140)=3.390, P =0.0014; * P ≤0.05, Bonferroni test, n =9 mice per group). ( d ) Survival is reduced in ad-MyoD-injected mice (Kaplan–Meier analysis, log-rank, P =0.0018). ad-MyoD (dashed line); ad-GFP (solid line); n =9 mice per group. ( e ) Western blotting shows that neither the mutant SOD1 ( f , hSOD1) nor the mouse SOD1 ( g , mSOD1) is altered following MyoD gene transfer ( n =4 samples per group). Data are presented as mean±s.e.m. Full size image Recent studies have demonstrated that muscle-specific transgenic expression of mutant SOD1 can cause muscle dysfunction [6] and motor neuron degeneration [5] in mice. Examination of tissue samples by western blotting showed that neither the mutant ( Fig. 2e,f ; full blot images, Supplementary Fig. 1 ) nor mouse SOD1 levels ( Fig. 2e,g ; full blot images, Supplementary Fig. 1 ) were altered in muscle by MyoD gene transfer, ruling out the possibility of SOD1 modulation in muscle by MyoD as a cause of disease acceleration in G93A mice. Also, the effect observed in G93A mice was disease-specific since similar treatment in non-transgenic littermates did not have any behavioural impact. Weekly assessment of these mice showed consistent weight gain over time ( Fig. 3a ) and their ability to stay on the rotarod for full 420 s over the course of the testing period ( Fig. 3b ). These mice remained healthy and did not show any behavioural abnormality even at 6 months following injection, showing that muscle-directed MyoD gene transfer itself was not toxic. 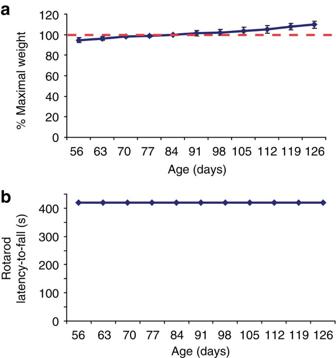Figure 3: Muscle-directed MyoD gene transfer is not harmful in non-transgenic littermates. Non-transgenic mice were injected with adenovirus containing MyoD construct (Ad-MyoD) combined with transient CD4+cell depletion (n=8 mice). These mice were behaviourally observed starting at 56 days of age. (a) Weekly assessment of these mice showed consistent weight gain over time. (b) Weekly rotarod assessment at 20 r.p.m. showed consistent ability of mice to stay on the rotating beam for full 420 s over the duration of testing. After this period the mice were no longer tested but continued being observed. These mice were healthy and did not show any behavioural abnormality even at 6 months following injection. Red dashed line denotes weight at 84 days of age set as 100%. Data are presented as mean±s.e.m. Figure 3: Muscle-directed MyoD gene transfer is not harmful in non-transgenic littermates. Non-transgenic mice were injected with adenovirus containing MyoD construct (Ad-MyoD) combined with transient CD4 + cell depletion ( n =8 mice). These mice were behaviourally observed starting at 56 days of age. ( a ) Weekly assessment of these mice showed consistent weight gain over time. ( b ) Weekly rotarod assessment at 20 r.p.m. showed consistent ability of mice to stay on the rotating beam for full 420 s over the duration of testing. After this period the mice were no longer tested but continued being observed. These mice were healthy and did not show any behavioural abnormality even at 6 months following injection. Red dashed line denotes weight at 84 days of age set as 100%. Data are presented as mean±s.e.m. Full size image Myogenin gene transfer improves rotarod performance In our second set of experiments, we injected the hindlimb muscles of adult male G93A mice with either ad-myogenin or ad-GFP. Human myogenin expression in the muscle following ad-myogenin injection was confirmed via qPCR ( Fig. 4a ; t -test, P <0.00001; n =9 mice per group). Comparison of rotarod performance between ad-myogenin and ad-GFP injected mice showed statistically significant treatment effect ( Fig. 4b , two-way ANOVA, F (1,186)=30.26; P <0.0001; n =9 mice per group). Bonferroni post-tests show statistically significant improvement in rotarod performance for ad-myogenin injected mice at 91 ( P <0.05), 98 ( P <0.05), 105 ( P <0.001) and 112 ( P <0.01) days of age. Myogenin overexpression however did not affect either the weight-loss profile ( Fig. 4c ) or survival ( Fig. 4d ). We did not measure the expression levels of hSOD1 in these groups of mice since the study from Cleveland group showed that the knockdown of mutant SOD1 does not affect the disease progression in the fALS mice [7] . 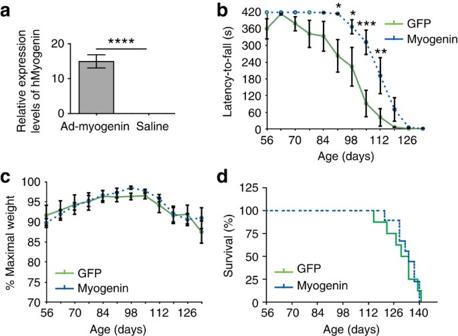Figure 4: Myogenin gene-transfer into Adult G93A hindlimb muscle improves rotarod performance. (a) Expression of human myogenin in the muscle following adenoviral construct injection was confirmed using quantitative real-time PCR (n=4 per group,t-test, ****P<0.00001). (b) Ad-myogenin-injected mice are able to remain on the rotarod for longer duration than ad-GFP-injected mice starting at 91 days of age (two-way ANOVA,F(1,140)=23.33,P≤0.0001; Bonferronipost hoctest; *P≤0.05; **P<0.01; ***P<0.001;n=9 mice per group). There was no difference in the weight-loss profile (c) and survival rate (d) between the two treatment groups. Ad-myogenin (dashed line); ad-GFP (solid line);n=9 mice per group. Data are presented as mean±s.e.m. Figure 4: Myogenin gene-transfer into Adult G93A hindlimb muscle improves rotarod performance. ( a ) Expression of human myogenin in the muscle following adenoviral construct injection was confirmed using quantitative real-time PCR ( n =4 per group, t -test, **** P <0.00001). ( b ) Ad-myogenin-injected mice are able to remain on the rotarod for longer duration than ad-GFP-injected mice starting at 91 days of age (two-way ANOVA, F (1,140)=23.33, P ≤0.0001; Bonferroni post hoc test; * P ≤0.05; ** P <0.01; *** P <0.001; n =9 mice per group). There was no difference in the weight-loss profile ( c ) and survival rate ( d ) between the two treatment groups. Ad-myogenin (dashed line); ad-GFP (solid line); n =9 mice per group. Data are presented as mean±s.e.m. Full size image Differential motor neuron degeneration In our two independent experiments, rotarod testing showed improvement in motor performance following myogenin gene transfer compared with GFP control mice while MyoD gene transfer worsened motor performance in G93A mice as the disease progressed in comparison to the GFP control group. To determine whether spinal cord motor neuron degeneration is affected by exogenous expression of MyoD and myogenin in muscle, ventral horn motor neurons in the lumbar spinal cord region (L3–L5) were counted stereologically using size-exclusion criteria [19] . We examined spinal cord samples from 100-day-old animals as these mice show significant motor neuron loss starting at 90-days of age [20] . Examination of cresyl violet-stained spinal cord sections showed decreased ventral horn staining pattern in ad-MyoD injected mice compared with ad-GFP-injected mice ( Fig. 5a versus b ). On the other hand, ventral horns of ad-myogenin injected mice showed increased staining pattern in the ventral horn compared with ad-GFP injected mice ( Fig. 5a versus c ). Under higher magnification, ad-MyoD-injected mice motor neurons displayed smaller cell body size compared with ad-GFP-injected mice ( Fig. 5d versus e ), suggesting increased atrophy. Spinal cord samples from ad-myogenin mice showed motor neurons that were larger and asymmetrical in shape compared with motor neurons in ad-GFP-injected mice, which were smaller and rounder in shape ( Fig. 5d versus f ). 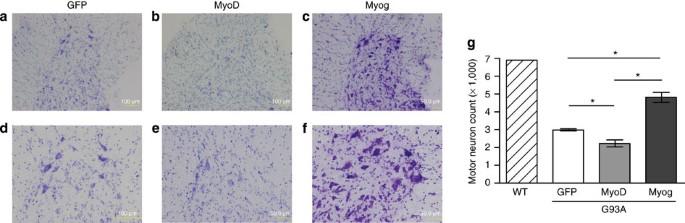Figure 5: Muscle gene transfer of either MyoD or myogenin differentially modulates spinal cord motor neuron degeneration in G93A mice. The impact of MyoD or myogenin muscle gene transfer on spinal cord motor neuron degeneration was determined by analysing lumbar spinal cord sample from 100-day-old mice. Examination of ventral horn motor neurons at lower magnification ( × 10) showed that compared with ad-GFP-injected G93A mice (a), motor neurons in ad-MyoD-injected G93A mice were sparsely distributed (b). Ad-myogenin-injected mice on the other hand showed greater number of motor neurons (c). Motor neuron morphology also seems to be affected by the treatment. Higher magnification images ( × 20) showed that in comparison to the ad-GFP-injected samples (d), motor neurons in ad-MyoD-injected mice were smaller (e). In contrast, motor neurons were less rounded and larger in ad-myogenin-injected mice (f). Stereological examination of spinal cord sections showed an impact of muscle-directed MyoD and myogenin gene transfer on motor neuron counts using size exclusion criteria (g). Ad-MyoD-injected mice showed 26% fewer motor neurons counted compared with ad-GFP-injected control mice (one-way ANOVA,P<0.0001; Tukey’spost hoctest, *P<0.05,n=5 samples per group). Ad-myogenin-injected mice on the other hand showed 66% more motor neuron counts compared with ad-GFP-injected mice (one-way ANOVA,P<0.0001; Tukey’spost hoctest, *P<0.001,n=5 samples per group). Statistically significant differences between the means are represented by different colours and asterisks (*). Data are presented as mean±s.e.m. WT (n=1) was not included in statistical analysis but shown as a benchmark (diagonal pattern).n=5 spinal cord samples per treatments (GFP, MyoD and Myog). Scale bars represent 100 μm. Figure 5: Muscle gene transfer of either MyoD or myogenin differentially modulates spinal cord motor neuron degeneration in G93A mice. The impact of MyoD or myogenin muscle gene transfer on spinal cord motor neuron degeneration was determined by analysing lumbar spinal cord sample from 100-day-old mice. Examination of ventral horn motor neurons at lower magnification ( × 10) showed that compared with ad-GFP-injected G93A mice ( a ), motor neurons in ad-MyoD-injected G93A mice were sparsely distributed ( b ). Ad-myogenin-injected mice on the other hand showed greater number of motor neurons ( c ). Motor neuron morphology also seems to be affected by the treatment. Higher magnification images ( × 20) showed that in comparison to the ad-GFP-injected samples ( d ), motor neurons in ad-MyoD-injected mice were smaller ( e ). In contrast, motor neurons were less rounded and larger in ad-myogenin-injected mice ( f ). Stereological examination of spinal cord sections showed an impact of muscle-directed MyoD and myogenin gene transfer on motor neuron counts using size exclusion criteria ( g ). Ad-MyoD-injected mice showed 26% fewer motor neurons counted compared with ad-GFP-injected control mice (one-way ANOVA, P <0.0001; Tukey’s post hoc test, * P <0.05, n =5 samples per group). Ad-myogenin-injected mice on the other hand showed 66% more motor neuron counts compared with ad-GFP-injected mice (one-way ANOVA, P <0.0001; Tukey’s post hoc test, * P <0.001, n =5 samples per group). Statistically significant differences between the means are represented by different colours and asterisks (*). Data are presented as mean±s.e.m. WT ( n =1) was not included in statistical analysis but shown as a benchmark (diagonal pattern). n =5 spinal cord samples per treatments (GFP, MyoD and Myog). Scale bars represent 100 μm. Full size image Stereological analysis of ventral horn motor neurons from 2 mm portion of lumbar region of spinal cord revealed that muscle-directed gene transfer of MyoD or myogenin had a treatment-dependent effect on the motor neuron count based on size exclusion criteria (cross-sectional area of >200 μm 2 ). Ad-MyoD-injected mice showed 26% fewer motor neurons counted compared with ad-GFP-injected control mice ( Fig. 5g , one-way ANOVA, P <0.0001; Tukey’s post-test, P <0.05; n =5 samples per group). On the other hand, ad-myogenin-injected mice showed 66% more motor neurons counted compared with ad-GFP-injected mice ( Fig. 5g , Tukey’s post-test, P <0.001; n =5 samples per group). The motor neuron count in ad-myogenin-injected mice is also greater than in ad-MyoD-injected mice (Tukey’s post-test, P <0.001; n =5 samples per group). Our results suggest that an exogenous expression of myogenin in muscle helps preserve spinal cord motor neurons while exogenous expression of MyoD in muscle enhances motor neuron degeneration in G93A mice. Differential muscle denervation Muscle denervation has been shown to precede motor neuron loss in G93A mice [21] , [22] . Furthermore, Bax deletion-mediated rescue of motor neurons failed to halt muscle endplate denervation [23] . To determine whether muscle endplate innervation pattern is modulated following MyoD or myogenin gene transfer, we stereologically examined muscle sections from 100-day-old experimental animals. Muscle sections were fluorescently labelled with rhodamine-conjugated α-bungarotoxin along with synaptophysin and neurofilament antibodies ( Fig. 6a ). Muscle innervation patterns were classified as ‘innervated’, ‘intermediate’ or ‘denervated’ according to the staining patterns ( Fig. 6a , also described in Methods). 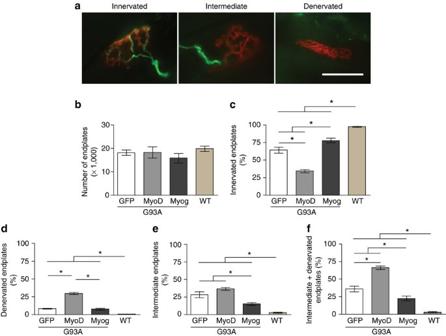Figure 6: Muscle gene transfer of either MyoD or myogenin differentially modulates muscle endplate innervation in G93A mice. Muscle endplates were examined in 100-day-old mice following muscle-directed gene transfer. (a) NMJ innervation patterns were categorized into one of three distinct patterns based on rhodamine-conjugated α-bungarotoxin (red) and synaptophysin (green) and neurofilament (green) staining patterns. (b) Stereological analysis of exhaustively sectioned muscle samples (n=4 muscles per treatment conditions (GFP, MyoD, Myog and WT)) did not show any difference in the total number of muscle endplates between groups. However, the proportions of innervated (c, one-way ANOVA,P<0.0001,n=4 samples per group), denervated (d, one-way ANOVA,P<0.0001,n=4 samples per group) and intermediate (e, one-way ANOVA,P<0.0001,n=4 samples per group) muscle endplates were significantly different between various treatment groups. Muscle innervation was increased in myogenin gene transfer group, whereas MyoD gene transfer decreased the proportion of innervated muscle endplates compared with GFP gene transfer mice (c, Tukey’spost hoctest; Myog versus GFP, *P<0.05,n=4 samples per group; MyoD versus GFP, *P<0.001,n=4 samples per group). The proportion of denervated endplates was significantly increased in ad-MyoD-injected mice (d, Tukey’spost hoctest; MyoD versus GFP, *P<0.001,n=4 samples per group) and myogenin gene transfer resulted in the reduction of intermediate muscle endplates (e, Tukey’spost hoctest, *P<0.05,n=4 samples per group). When the proportions of denervated and intermediate endplates were combined, there was a clear treatment-dependent effect between all the groups (f, one-way ANOVA,P<0.0001,n=4 samples per group). Following one-way ANOVA, multiple comparison test was performed using Tukey’s test. Different coloured bars and asterisks (*) represent statistically significant differences between the means. Data are presented as mean±s.e.m. Scale bar represents 25 μm. Figure 6: Muscle gene transfer of either MyoD or myogenin differentially modulates muscle endplate innervation in G93A mice. Muscle endplates were examined in 100-day-old mice following muscle-directed gene transfer. ( a ) NMJ innervation patterns were categorized into one of three distinct patterns based on rhodamine-conjugated α-bungarotoxin (red) and synaptophysin (green) and neurofilament (green) staining patterns. ( b ) Stereological analysis of exhaustively sectioned muscle samples ( n =4 muscles per treatment conditions (GFP, MyoD, Myog and WT)) did not show any difference in the total number of muscle endplates between groups. However, the proportions of innervated ( c , one-way ANOVA, P <0.0001, n =4 samples per group), denervated ( d , one-way ANOVA, P <0.0001, n =4 samples per group) and intermediate ( e , one-way ANOVA, P <0.0001, n =4 samples per group) muscle endplates were significantly different between various treatment groups. Muscle innervation was increased in myogenin gene transfer group, whereas MyoD gene transfer decreased the proportion of innervated muscle endplates compared with GFP gene transfer mice ( c , Tukey’s post hoc test; Myog versus GFP, * P <0.05, n =4 samples per group; MyoD versus GFP, * P <0.001, n =4 samples per group). The proportion of denervated endplates was significantly increased in ad-MyoD-injected mice ( d , Tukey’s post hoc test; MyoD versus GFP, * P <0.001, n =4 samples per group) and myogenin gene transfer resulted in the reduction of intermediate muscle endplates ( e , Tukey’s post hoc test, * P <0.05, n =4 samples per group). When the proportions of denervated and intermediate endplates were combined, there was a clear treatment-dependent effect between all the groups ( f , one-way ANOVA, P <0.0001, n =4 samples per group). Following one-way ANOVA, multiple comparison test was performed using Tukey’s test. Different coloured bars and asterisks (*) represent statistically significant differences between the means. Data are presented as mean±s.e.m. Scale bar represents 25 μm. Full size image Stereological analysis of muscle endplates labelled with α-bungarotoxin showed that the total number of muscle endplates per muscle was not different between various treatment groups ( Fig. 6b ). However, there was a statistically significant treatment-dependent effect on the number of innervated muscle endplates ( Fig. 6c , One-way ANOVA, F =44.12, P <0.0001; n =4 samples per group). A greater proportion of muscle endplates were innervated in ad-myogenin injected animals compared with ad-GFP injected mice ( Fig. 6c , Tukey’s post-test, P <0.05; n =4 samples per group). On the other hand, there was a significant reduction in the proportion of innervated muscle endplates in ad-MyoD injected mice compared with ad-GFP injected mice ( Fig. 6c , Tukey’s post-test, P <0.001; n =4 samples per group). Examination of denervated and intermediate endplates yielded mixed results. A higher proportion of denervated endplates were observed for the ad-MyoD-injected animals compared with the ad-GFP- and ad-myogenin-injected mice. ( Fig. 6d , one-way ANOVA, F =112.6, P <0.0001, n =4 samples per group; Tukey’s post-test, MyoD versus GFP: P <0.001, n =4 samples per group; myogenin versus MyoD: P <0.001, n =4 samples per group). The denervation pattern was not statistically different between ad-myogenin- and ad-GFP-injected animals ( Fig. 6d ). On the other hand, the proportion of intermediate endplates for ad-myogenin-injected animals showed statistically significant reduction in comparison to either ad-MyoD- or ad-GFP-injected mice ( Fig. 6e , one-way ANOVA, F =13.54, P <0.0019; Tukey’s post-test, myogenin versus GFP: P <0.05, n =4 samples per group; myogenin versus MyoD: P <0.01, n =4 samples per group). There was no statistical difference in intermediate endplate proportions between ad-MyoD- and ad-GFP-injected mice ( Fig. 6e ). When the proportions of intermediate and denervated muscle endplates were combined, there was a clear treatment-dependent effect ( Fig. 6f , one-way ANOVA, F =43.5, P <0.0001, n =4 samples per group). Compared with the ad-GFP-injected group, the proportion of intermediate and denervated endplates was significantly reduced in the ad-myogenin-injected animals ( Fig. 6f , Tukey’s post-test, myogenin versus GFP: P <0.05, n =4 samples per group) and was significantly increased in ad-MyoD-injected animals ( Fig. 6f , Tukey’s post-test MyoD versus GFP: P <0.001, n =4 samples per group). Postnatal gene expression alters muscle phenotype The influence of muscle-directed MyoD and myogenin gene transfer on motor neuron loss and muscle endplate denervation suggests that ensuing modification of muscle properties may influence neuromuscular pathology in G93A mice. It has been shown that myogenin expression induces increased oxidative capacity in pre-existing muscle fibres [14] , [15] Quantitative real-time PCR (qPCR) shows differential expression of myosin heavy chain isoforms following gene transfer. Two weeks post-injection, ad-myogenin-injected muscle samples show increased expression of myh2 (MyHC IIa gene) ( Fig. 7a ; one-way ANOVA, P =0.028; Tukey’s post-test, ad-myogenin versus saline, P <0.05; n =4 samples per group). On the other hand, ad-MyoD-injected muscle sample show increased expression of myh4 (MyHC IIb gene) ( Fig. 7a ; one-way ANOVA, P =0.0083; Tukey’s post-test, ad-MyoD versus saline, P <0.05, n =4 samples per group; ad-MyoD versus ad-myogenin, P <0.01, n =4 samples per group). The expression levels for myh7 (MyHC I gene) was not statistically different between groups ( Fig. 7a ). Type IIa fast fibres are more oxidative than type IIb faster fibres. It has been shown that type IIb muscle fibres are preferentially denervated in G93A mice [24] . Therefore, oxidative muscle fibre composition in the muscle was assessed using succinic dehydrogenase (SDH) histochemistry. 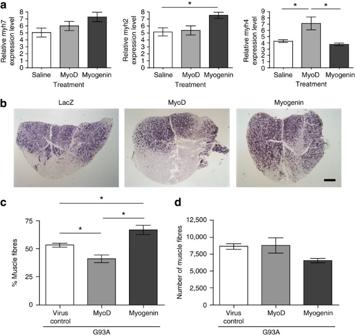Figure 7: Oxidative muscle phenotype in G93A mice is reorganized following postnatal gene transfer. (a) Expression levels for various myosin heavy chain isoforms were examined in muscle samples injected with ad-MyoD, ad-myogenin or saline using qPCR. Two weeks following injection, ad-myogenin-injected samples show increased expression formyh2(one-way ANOVA,P=0.028; Tukey’s post test, ad-myogenin versus saline, *P<0.05,n=4 samples per group). The difference in the expression levels formyh7was not statistically significant between treatments. On the other hand, ad-MyoD-injected samples show highermyh4expression level (one-way ANOVA,P=0.0083; Tukey’s post-test, ad-MyoD versus saline, *P<0.05,n=4 samples per group; ad-MyoD versus ad-Myogenin, *P<0.01,n=4 samples per group). (b) Transverse muscle sections from 100-day-old mice were histochemically stained for SDH in order to identify oxidative muscle fibres. (c) Stereological analysis of muscle samples from 100-day-old animals show increased proportion of oxidative muscle fibres (SDH-positive) in ad-myogenin-injected animals (one-way ANOVA,F=16.6,P<0.0002; Tukey’s post-test, ad-myogenin versus virus control, *P<0.5,n=6 samples per group; ad-myogenin versus ad-MyoD, *P<0.001,n=6 samples per group). On the other hand, ad-MyoD-injected muscle sample showed reduction in the proportion of SDH-positive oxidative muscle fibres (Tukey’s post-test, ad-MyoD versus virus control, *P<0.05,n=6 samples per group). (d) Total number of muscle fibres was not statistically different between treatment groups, suggesting remodeling of muscle oxidative phenotype by MyoD and myogenin gene transfer. Asterisks (*) denote statistical difference. Data are presented as mean±s.e.m. Scale bar represents 500 μm. Figure 7: Oxidative muscle phenotype in G93A mice is reorganized following postnatal gene transfer. ( a ) Expression levels for various myosin heavy chain isoforms were examined in muscle samples injected with ad-MyoD, ad-myogenin or saline using qPCR. Two weeks following injection, ad-myogenin-injected samples show increased expression for myh2 (one-way ANOVA, P =0.028; Tukey’s post test, ad-myogenin versus saline, * P <0.05, n =4 samples per group). The difference in the expression levels for myh7 was not statistically significant between treatments. On the other hand, ad-MyoD-injected samples show higher myh4 expression level (one-way ANOVA, P =0.0083; Tukey’s post-test, ad-MyoD versus saline, * P <0.05, n =4 samples per group; ad-MyoD versus ad-Myogenin, * P <0.01, n =4 samples per group). ( b ) Transverse muscle sections from 100-day-old mice were histochemically stained for SDH in order to identify oxidative muscle fibres. ( c ) Stereological analysis of muscle samples from 100-day-old animals show increased proportion of oxidative muscle fibres (SDH-positive) in ad-myogenin-injected animals (one-way ANOVA, F =16.6, P <0.0002; Tukey’s post-test, ad-myogenin versus virus control, * P <0.5, n =6 samples per group; ad-myogenin versus ad-MyoD, * P <0.001, n =6 samples per group). On the other hand, ad-MyoD-injected muscle sample showed reduction in the proportion of SDH-positive oxidative muscle fibres (Tukey’s post-test, ad-MyoD versus virus control, * P <0.05, n =6 samples per group). ( d ) Total number of muscle fibres was not statistically different between treatment groups, suggesting remodeling of muscle oxidative phenotype by MyoD and myogenin gene transfer. Asterisks (*) denote statistical difference. Data are presented as mean±s.e.m. Scale bar represents 500 μm. Full size image Histochemical examination of transverse gastrocnemius muscle sections from 100-day-old mice shows differences in the distribution of oxidative fibres between the treatment groups. Ad-myogenin-treated muscles show a uniform distribution of oxidative muscle fibres as indicated by darkly stained muscle fibres compared with virus control (samples injected with either ad-GFP or ad-Lacz) and MyoD muscle samples ( Fig. 7b ). Stereological count of SDH stained muscle fibres in 100-day-old experimental mice show that the oxidative fibres account for ~67% of total muscle fibres in the gastrocnemius injected with ad-myogenin ( Fig. 7c , n =6). In the virus control muscle samples, SDH positive muscle fibres represent ~53% of the total muscle fibres ( Fig. 7c , n =6). On the other hand, MyoD-treated muscle samples show only 41% of the muscle fibres that are stained positively for SDH, fewer oxidative muscle fibres compared with virus control ( Fig. 7c , n =6). These values were statistically different from each other (one-way ANOVA, F =16.6, P =0.0002; virus control versus ad-myogenin, Tukey’s post-test, P <0.05, n =6 samples per group; virus control versus ad-MyoD, Tukey’s post-test, P <0.05, n =6 samples per group; ad-myogenin versus ad-MyoD, Tukey’s post-test, P <0.001, n =6 samples per group). The total number of muscle fibres was not statistically different between treatment groups in the 100-day-old mice ( Fig. 7d ). PGC-1α does not improve survival or motor performance To examine whether enhanced mitochondrial biogenesis in muscle by PGC-1α overexpression improves disease progression in the G93A SOD1 fALS mouse model, we crossed G93A mice with transgenic mice overexpressing PGC-1α under the control of muscle creatine kinase (MCK-PCG-1α mice). PGC-1α is a potent metabolic regulator in the muscle and an overexpression of PGC-1α in muscle was reported to cause increased mitochondrial protein and oxidative capacity [16] , [25] . In mice over-expressing PGC-1α in muscle, mitochondrial activity in the gastrocnemius of G93A/MCK-PGC-1α mice was increased as indicated by increased SDH staining in the muscle ( Fig. 8a ). G93A and G93A/MCK-PGC-1α male mice were longitudinally observed to examine the effect of PGC-1α overexpression in muscle on the disease progression. We did not observe any difference in the survival rate ( Fig. 8b , G93A: 163 days versus G93A/MCK-PGC-1α: 162 days) or progressive weight loss ( Fig. 8c ) between G93A and G93A/MCK-PGC-1α mice. Motor function was also longitudinally assessed in these mice using various motor function tests. Rotarod analysis demonstrated a genotypic difference between the two genotypic groups ( Fig. 8d , two-way ANOVA, P <0.0001; n =9 SOD1; n =7 SOD1/MCK-PGC-1α). Bonferroni post hoc analysis showed that G93A/MCK-PGC-1α mice performed worse at 112 ( P <0.001), 119 ( P <0.001), 126 ( P <0.001) and 133 ( P <0.001) day time-points ( Fig. 8d ). Paw grip strength was tested using grip strength meter and paw grip endurance (PaGE) test ( Fig. 8e,f , respectively). Two-way ANOVA showed significant genotype effect on the paw grip strength ( Fig. 8e , Two-way ANOVA, P <0.0001, n =9 G93A; n =7 G93A/MCK-PGC-1α). Bonferroni post hoc analysis showed that G93A/MCK-PGC-1α mice performed worse at 98-day time-point ( Fig. 8e , P<0.05, n=9 G93A; n=7 G93A/MCK-PGC-1α). PaGE test also showed significant genotype effect ( Fig. 8f , Two-way ANOVA, P =0.0082, n =9 G93A; n =7 G93A/MCK-PGC-1α). However, there was no statistically significant difference in PaGE between the two genotypes during any of the time points observed during the course of the disease ( Fig. 8f , Bonferroni post-test, n =9 G93A; n =7 G93A/MCK-PGC-1α). Therefore, enhancement of mitochondrial biogenesis by constitutive muscle expression of PGC-1α did not affect survival but seemed to have a negative effect on the motor function. 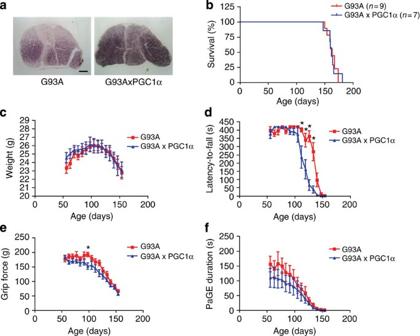Figure 8: PGC-1α-mediated increase in the muscle oxidative phenotype does not improve survival or motor function in G93A mice. G93A mice were mated with MCK-PGC-1α mice to examine the effect of enhanced mitochondrial biogenesis in the muscle on disease progression. (a) Gastrocnemius muscle from G93A/MCK-PGC-1α mouse shows higher SDH staining than S93A mouse, demonstrating increased mitochondrial activity in the presence of PGC-1α transgene (scale=500 μm). (b) Survival analysis and (c) weekly weight measures (two-way ANOVA,n=9 G93A;n=7 G93A/MCK-PGC-1α) did not show a genotypic difference between the two groups. (c) Motor function was examined in these mice using the rotarod apparatus. The difference in the rotarod latency-to-fall values between the two groups were statistically significant (two-way ANOVA,P<0.0001,n=9 G93A;n=7 G93A/MCK-PGC-1α). Bonferroni test shows G93A/MCK-PGC-1α mice performed worse at 112 (*P<0.001), 119 (*P<0.001), 126 (*P<0.001) and 133 (*P<0.001) day time-points. Paw grip strength was longitudinally examined using grip strength meter (e) and paw grip endurance test (PaGE,f). Statistical analysis revealed a significant genotype effect for both the grip strength and PaGE (e,f, respectively; two-way ANOVA;e:P<0.0001;f:P=0.0082,n=9 G93A;n=7 G93A/MCK-PGC-1α). Bonferroni post-test shows that SOD1/PGC1-α mice performed significantly worse at 98-day time-point for the grip strength (e, Bonferroni post-test, *P<0.05,n=9 G93A;n=7 G93A/MCK-PGC-1α). However, there was no difference between the genotypes at any of the time-points for the PaGE test (f). Therefore, enhancement of mitochondrial biogenesis in the muscle via PGC-1α overexpression did not improve survival but worsened motor function in G93A mice. Asterisks (*) denote statistical difference. Data are presented as mean±s.e.m. Figure 8: PGC-1α-mediated increase in the muscle oxidative phenotype does not improve survival or motor function in G93A mice. G93A mice were mated with MCK-PGC-1α mice to examine the effect of enhanced mitochondrial biogenesis in the muscle on disease progression. ( a ) Gastrocnemius muscle from G93A/MCK-PGC-1α mouse shows higher SDH staining than S93A mouse, demonstrating increased mitochondrial activity in the presence of PGC-1α transgene (scale=500 μm). ( b ) Survival analysis and ( c ) weekly weight measures (two-way ANOVA, n =9 G93A; n =7 G93A/MCK-PGC-1α) did not show a genotypic difference between the two groups. ( c ) Motor function was examined in these mice using the rotarod apparatus. The difference in the rotarod latency-to-fall values between the two groups were statistically significant (two-way ANOVA, P <0.0001, n =9 G93A; n =7 G93A/MCK-PGC-1α). Bonferroni test shows G93A/MCK-PGC-1α mice performed worse at 112 (* P <0.001), 119 (* P <0.001), 126 (* P <0.001) and 133 (* P <0.001) day time-points. Paw grip strength was longitudinally examined using grip strength meter ( e ) and paw grip endurance test (PaGE, f ). Statistical analysis revealed a significant genotype effect for both the grip strength and PaGE ( e , f , respectively; two-way ANOVA; e : P <0.0001; f : P =0.0082, n =9 G93A; n =7 G93A/MCK-PGC-1α). Bonferroni post-test shows that SOD1/PGC1-α mice performed significantly worse at 98-day time-point for the grip strength ( e , Bonferroni post-test, * P <0.05, n =9 G93A; n =7 G93A/MCK-PGC-1α). However, there was no difference between the genotypes at any of the time-points for the PaGE test ( f ). Therefore, enhancement of mitochondrial biogenesis in the muscle via PGC-1α overexpression did not improve survival but worsened motor function in G93A mice. Asterisks (*) denote statistical difference. Data are presented as mean±s.e.m. Full size image Our hypothesis was based on experimental evidence suggesting a possible effect of muscle phenotype on the disease progression; fast muscle fibres and motor units are seemingly selectively vulnerable in ALS, while slow muscle fibres, which have greater oxidative capacity, seem to be relatively preserved in the disease [1] , [2] , [3] , [4] , [24] . To test our hypothesis, we used viral-mediated postnatal expression of two distinct muscle-specific basic helix–loop–helix transcription factors to directly examine whether muscle phenotype influences disease progression in G93A mouse model of ALS. MyoD and myogenin along with MRF4 and myf5 form a family of myogenic regulatory factors (MRF) that are involved in muscle development and differentiation [26] . MyoD and myogenin govern differential muscle gene expression [27] . In the adult muscle, MyoD is highly expressed in fast muscle fibres [11] , [12] and regulates fast muscle development [12] . On the other hand, myogenin is highly expressed in slow muscle fibres [11] and its expression increases oxidative metabolism in the muscle [14] , [15] . In this study, we used adenovirus to exogenously express MyoD and myogenin in the hindlimb muscles of adult G93A mice to examine whether MyoD and myogenin expression in the adult muscle can impact disease progression in an ALS mouse model. Lack of X-gal staining in the spinal cord following injection of adenovirus expressing LacZ into the muscle suggests that that the adenovirus is not retrogradely taken up by the motor neurons and the gene expression is confined to the muscle in our study. Our findings show that exogenous expression of myogenin in adult muscle results in increased motor neuron count and muscle innervation. On the other hand, exogenous expression of MyoD in the adult muscle results in reduced motor neuron count, muscle innervation and survival. We have previously shown that MyoD expression is decreased in the muscle of G93A mice at 27 days of age [28] . Our current finding suggests that this early decrease in MyoD expression may be a protective compensation. We are currently testing this hypothesis by postnatally knocking down MyoD in the G93A mice. Ad-myogenin-injected muscle samples showed higher expression of MyHC IIa gene myh2. On the other hand, ad-MyoD-injected muscle samples showed higher expression of MyHC IIb gene myh4. Correspondingly, there was an increase in the proportion of muscle fibres that were strongly stained for SDH in animals injected with ad-myogenin. The total number of muscle fibres between the treatment groups in our study was not statistically different, suggesting an oxidative muscle phenotype conversion by myogenin gene transfer in adult mice. These findings are in agreement with past studies that showed muscle fibre type switching with MyoD and myogenin gene transfer. Myogenin gene transfer has been shown to convert glycolytic muscle fibres to oxidative muscle fibres [14] , [15] . MyoD gene transfer has shown to impart type IIb muscle fibre under denervation condition [13] . Our data suggest that MyoD and myogenin gene transfer in the G93A mice at presymptomatic age modulates gene expression and modifies muscle phenotype. The differential effect on neuropathology at 100 days of age in our study suggests that the disease progression can be altered by postnatal muscle phenotype modification. However, the exact physiological changes responsible for mediating the effect in our study remain unclear. More in-depth analysis of physiological changes occurring in the muscle following MyoD and myogenin induction may provide insight into physiological mechanisms affecting NMJ denervation in ALS. An alternative approach using constitutive overexpression of transgenic PGC-1α to induce an increased oxidative phenotype did not improve survival and worsened motor function in these mice. A similar finding was also reported for the G37R SOD1 mouse model [29] . The similar findings between G93A and G37R mouse models of ALS in response to transgenic expression of PGC1-a confirms our methodology and suggests that the MyoD and myogenin findings are unlikely to be due to model differences. The differential clinical outcome in the fALS mouse model between myogenin- and PGC-1α-mediated muscle remodeling despite the enhanced oxidative phenotype for both factors may be due to differential gene regulation between myogenin and PGC-1α. For example, it has been shown that AICAR-mediated increase in muscle expression of mitochondrial proteins requires PGC-1α (ref. 30 ). However, myogenin expression remains unchanged despite increased PGC-1α expression in response to AICAR treatment [31] . Another possibility is that myogenin expression is virally induced in postnatal muscle, whereas PGC-1α is transgenically expressed. Transgenic expression of PGC-1α may induce developmental compensatory gene regulation, which may be the reason behind the differential effect on the disease progression in the G93A mice. It has been shown that muscle denervation precedes motor neuron loss in fALS mouse models and ALS patients [21] , [22] , [32] . Although, MyoD and myogenin have been shown to activate acetylcholine receptor expression in the muscle [33] , [34] , [35] , [36] , we did not observe any difference in the total number of α-bungarotoxin-bound actetylcholine receptors between the treatment groups. Findings by Williams et al. [37] showed that muscle-specific microRNA-206 (miR-206), which is also enriched in slow muscle, is important for muscle reinnervation process and developmental knockout of miR-206 in G93A mice accelerates disease progression by delaying muscle reinnervation in these mice. Myogenin is a transcriptional regulator of miR-206 (ref. 38 ); therefore, an increase in myogenin expression could enhance muscle reinnervation process in these mice. However, it is intriguing that muscle denervation is increased in response to MyoD gene transfer since MyoD can also activate miR-206 (ref. 37 ). Our finding seems to suggest a differential role of MyoD and myogenin in muscle endplate innervation/denervation process in adult G93A mice and further study will be necessary to determine the role of MyoD and myogenin in the muscle denervation process in the ALS. Findings from our study provide a potential insight into the role of exercise in ALS. Myogenin and MyoD expression pattern in response to exercise is quite complex and depends on the type of exercise [26] , [39] . For instance, MyoD expression in muscle is highest following high-intensity eccentric exercises [39] , [40] . On the other hand, in vivo expression of myogenin is closely correlated with the duration of moderate exercise [39] , [41] , [42] . However, some of the exercise studies show that both the MyoD and myogenin levels are elevated following either resistance or endurance training [26] . In cases of strength exercises such as eccentric or resistance exercises that cause muscle damage and repair, MyoD and myogenin are both elevated [26] . The expression of MyoD can be quite dynamic as well depending on the type of exercise [39] . The role of exercise has been controversial due to its seemingly conflicting effects on ALS progression reported by various groups. In human subjects, various groups have concluded that exercise is either beneficial or has no benefit [43] , [44] , [45] , [46] . In contrast, a number of retrospective studies in ALS patients have highlighted strenuous athletics or activities as potential risk factors for ALS [47] , [48] . Studies in ALS mouse models show that moderate exercise delays motor decline [49] , [50] , while high-intensity endurance exercise hastens disease progression [51] . Our findings suggest that strenuous exercise or activity that enhances muscle expresssion of MyoD will likely exacerbate ALS disease progression. Additionally, the beneficial exercises for ALS patients would be the ones that enhance myogenin expression in the muscle. It is worth noting that IGF-1, which has shown benefit in G93A mice [8] , [52] , increases myogenin expression in muscle [53] , [54] . Our findings need to be confirmed using other mouse models of fALS to determine whether the observations made in our study may have implications for disease management in ALS patients. A number of studies have now suggested extraneuronal cells influence motor neuron survival in ALS [55] , [56] , [57] , [58] , [59] . However, the potential role of muscle in pathogenesis has been controversial [5] , [6] , [7] , [29] . Our experimental evidence demonstrates that postnatal muscle expression of myogenic factors, MyoD and myogenin, modulates spinal cord motor neuron degeneration, muscle denervation and survival in the G93A SOD1 fALS mouse model. Unlike the beneficial effects of myogenin expression in muscle, constitutive overexpression of PGC1α in the muscle of G93A mice did not improve the outcome in this fALS model, consistent with a recent report. However, this finding does not reflect the potential benefits of postnatal modification of muscle in ALS using other factors, and may reflect pleotropic effects of this transcriptional modifier in addition to increases in muscle oxidative function. Our findings suggest that muscle phenotype moderately influences ALS pathogenesis in the G93A mouse model of ALS. However, this may be due to localized viral injection limited to a small muscle group in our study. A more systemic induction may lead to an increase in therapeutic benefit. Also, it will be necessary to examine other mouse models of fALS to further validate the role of MyoD and myogenin in ALS pathology. Further work in identifying key muscle biochemical pathways by which MyoD and myogenin influence disease progression may lead to effective muscle-directed treatments for ALS. Animals High copy number B6/SJL G93A mice (male and female mice, 50 days of age) were obtained from Jackson Laboratory (Bar Harbor, ME, USA) and bred and maintained in our animal colony. Mice were maintained on a 12-h light/dark cycle with free access to food and water. For PGC-1α muscle overexpression study, B6 congenic G93A mice (Jackson Laboratory) were crossed to B6 congenic MCK-PGC-1α mice (Jackson Laboratory) to generate G93A/MCK-PGC-1α mice. Male mice were used for this study and the genotyping was performed using genomic DNA, as suggested by the Jackson Laboratory genotyping protocol. Mice were killed by decapitation at end-stage and spinal cord and hindlimb muscles were quickly dissected. Dissected samples were either flash-frozen for biochemical analysis or immersion-fixed in 4% paraformaldehyde for immunohistological analysis. Muscle samples were fixed for 2 h at 4 °C and transferred to 30% sucrose solution for 2 h prior to freezing in OCT (TissueTek). All animal protocols were approved by the Animal Care Committee at the University of British Columbia. Antibodies and reagents The following antibodies were used in this study: mutant hSOD1 (1:1,000) (Novocastra NCL-SOD1, Vector Laboratories; Burlingame, CA, USA); CD4 antibody (100 μg per injection) (eBioscience Inc.; San Diego, CA, USA; Cat. No. 16-0041); mouse SOD1 (1:1,000) (Biosensis Pty Ltd.; Thebarton, South Australia; Cat. No. R-126-100); GAPDH (1:1,000) (Chemicon; Billerica, MA, USA; Cat. No. MAB374); rhodamine-conjugated α-bungarotoxin (1:500) (Invitrogen; Cat. No. B13423); synaptophysin (1:500) (Millipore, Billerica, MA, USA; Cat. No. MAB368); neurofilament (1:500) (Covance, Princeton, NJ, USA; Cat. No. SMI-32R). Adenoviral constructs were obtained from Vector Biolabs (Philadelphia, PA, USA). Sodium succinate, sodium phosphate (monbasic and dibasic), nitrobluetetrazolium tablets and normal goat serum were obtained from Sigma. Adenoviral injections Male mice were injected at 30 days of age with replication-incompetent adenovirus (AV) containing GFP, human MyoD or human myogenin construct under the control of cytomegalovirus promoter. Adenoviral constructs were obtained from Vector Biolab. A total of 5 × 10 [8] plaque-forming units were injected per site in the hindlimb (gastrocnemius, tibialis anterior, hamstring and quadriceps) combined with transient depletion of CD4+ cells using commercially available functional grade CD4 antibody (eBioscience) to enhance gene transfer and expression [60] . CD4 antibody (100 μg) was injected intraperitoneally 3 days and 1 day prior to intramuscular adenoviral injections followed by intraperitoneal injections of CD4 antibody 1 day and 3 days post AV injection. Mice were anesthetized using isofluorane prior to AV injections. Following injections, mice were monitored daily following recovery. None of the treated mice showed any adverse reactions to combined treatments of adenovirus and CD4 antibody. Behavioural tests Mice were trained at 47 days of age on the rotarod (UGO Basile, Italy) for a maximum duration of 7 min (420 s) at 20 r.p.m. Mice were weighed and tested weekly on the rotarod (UGO Basile) and grip test (Columbus Instruments) starting at 57 days of age. Mice were tested on the rotarod for maxium duration of 7 min (420 s). If the animal fell off prior to the maximal duration, they were tested for four trials in total and the maximal duration was recorded. Grip strength measurement was repeated six times per session and the average value was recorded. Quantitative real-time PCR Muscle samples were dissected and stored in −20°C until processed (Qiagen, Valencia, CA, USA). RNA extraction was performed using RNeasy Fibrous Tissue Midi Kit (Qiagen). cDNAs were generated using SuperScript VILO cDNA Synthesis Kit using 5 μg RNA input (Life Technologies, Carlsbad, CA, USA). Quantitative PCR was performed using the StepOne Plus Real-Time PCR system (Life Technologies) using 5 ng cDNA input per well. Fast SYBR Green Master Mix (Life Technologies) was used for all qPCR. Primer sequences were generated using either Primer Express 3.0 (Life Technologies) or PrimerQuest (IDT, Coralville, IA, USA). The primers were obtained from IDT. The sequences for the primers used in the study are listed in Table 1 . Gene expression levels are measured by real-time qPCR and expressed relative to the house-keeping genes GAPDH and HPRT. Table 1 List of primer sequences used for qPCR. Full size table Muscle endplate immunofluorescence Muscle sections were outlined using PAP pen (Research Products International) and incubated with rhodamine-conjugated α-bungarotoxin (1:500; Invitrogen) for 30 min at room temperature (RT). The sections were rinsed in 1 × TBS and fixed in ice-cold (−20 °C) MeOH for 10 min. The sections were rinsed with 1 × TBS and blocked with 3% normal goat serum in TBS for 30 min at RTThe sections were incubated with synaptophysin (1:500) and neurofilament (1:500) antibodies for 1 h at RT. The sections were rinsed with 1 × TBS and incubated with Alexafluor 488-conjugated secondary (goat anti-mouse, Invitrogen) for 1 h at RT. The sections were dehydrated in 100% EtOH and rinsed in Xylenes to remove PAP pen. The sections were rehydrated and cover-slipped using ProlongGold (Invitrogen). SDH staining SDH staining was performed according to SDH staining protocol obtained from Washington University muscle histology lab ( http://neuromuscular.wustl.edu/pathol/histol/sdh.htm ). Briefly, transverse 12-μm muscle sections were mounted on Super Frost microscope slides (Fisher Scientific). Sections were outlined with PAP pen (Research Products International) and incubated in buffer solution (20 mM phosphate buffer, 7.5% sucrose, 0.027% sodium succinate and 10 mg nitrobluetetrazoleum) for 45 min at RT. The sections were dehydrated and then briefly rinsed in 30, 60 and 90% acetone in ddH 2 O in ascending and descending order, rinsed in H 2 O, air-dried and cover-slipped using VectaMount (Vector Labs). X-gal staining Muscle samples were snap-frozen in liquid N 2 and sectioned at 16 um thickness and mounted on Superfrost microscope slides (Fisher). Briefly, the muscle sections were outlined with PAP pen and fixed at RT with 0.2% glutaraldehyde in TBS for 10 min. The sections were rinsed thrice with TBS and once with LacZ wash buffer (2 mM MgCl2, 0.1% sodium deoxycholate, 0.2% Nonidet, in 0.1 M phosphate buffer, pH 7) for 10 min. The sections were then stained overnight in LacZ staining solution (LacZ wash buffer, 1 mg ml −1 X-gal, potassium ferrocyanide, potassium ferricyanide). Stained muscle sections were fixed in 4% paraformaldehyde in TBS for 10 min and rinsed thrice in TBS. The sections were serially dehydrated in EtOH, cleared in xylenes and cover-slipped with DPX mounting medium. Intact spinal cord samples were immersion-fixed in 1% paraformaldehyde/0.2% glutaraldehyde in TBS for 30 min at RT. Spinal cords were then rinsed thrice in LacZ wash buffer (15 min each) and stained overnight at RT in LacZ staining solution. Stained spinal cord was fixed overnight at 4 °C in 4% paraformaldehyde/TBS. The fixed spinal cord was rinsed thrice in TBS (15 min each). The spinal cord was then embedded in 1.5% agar and sectioned using vibratome and mounted on Superfrost microscope slides. The mounted sections were dried overnight, cleared in xylenes and cover-slipped with DPX mounting medium. Cresyl violet staining Briefly, sequential lumbar sections were mounted on slides, dried overnight and stained with 0.5% cresyl violet for 6 min followed by dehydration with a graded series of ethanol solutions (70, 85, 90 and 100% for 2 min each). The slides were then treated with CitriSolv (Fisher, Tustin, CA, USA) for 2 min, followed by xylene for 10 min and cover-slipped with Cytoseal 60 (Richard-Allan Scientific, Kalamazoo, MI, USA). Western blotting Muscle samples were homogenized in lysis buffer (20 mM NaF, 1 mM Sodium Vanadate, 0.5% Triton X-100, 0.1% SDS and protease inhibitor cocktail (10 μl ml −1 ; Sigma, P8340) in 1 × TBS). Protein quantities were determined using Qubit quantitation platform (Invitrogen). Samples were electrophoresed using the Novex pre-cast gel system (Biorad), transferred to nitrocellulose (Protran, Schleicher and Schuell, Dassel, Germany) and subjected to immunoblotting. Band density was analysed using Quantity One software (Biorad, Mississauga, ON, USA). GAPDH (Millipore) was used as loading control. Precision Plus Protein Dual Colour Standards (Biorad) was used to determine the molecular weight sizing of protein bands. Tissue imaging Sections were observed using a Zeiss AxioPlan 2 microscope and images captured using a Coolsnap HQ camera (Photometrics, Tucson, AZ, USA) and MetaMorph software version 6.2r4 (Universal Imaging Corporation, Downingtown, PA, USA). Quantification of alpha motor neurons Spinal cords were dissected and isolated, immersed in paraformaldehyde overnight at 4 °C and then cryoprotected in 30% sucrose solution in TBS overnight at 4 °C. The lumbar spinal cord was then frozen in OCT compound (Sakura Finetek, Torrance, CA) and stored at −80 °C until sectioned. The tissue was cut in coronal 50-μm-thick consecutive sections and directly mounted on to Super Frost slides (Fisher Scientific). Stereological quantification of motorneurons was carried out on a series of cresyl violet-stained lumbar sections (every third lumbar section) with a total of 14 sections per mouse used in our calculations. Alpha motorneurons were selected based on morphology and size-exclusion criteria (area≥200 mm 2 ). A total estimated number of alpha motorneurons in the ventral horn per spinal cord was obtained using the Optical Fractionator Probe in StereoInvestigator 9.01, a morphometry and stereology software package (MicroBrightField, Colchester, VT, USA). Ventral horns were first delineated with a Zeiss × 2.5 objective and then cells were counted using a × 40 objective on a Zeiss Imager M2 microscope with a motorized computer-controlled stage (Ludl Electronics, Hawthorne, NY, USA) and a Microbrightfield Digital CCD video camera (MicroBrightField). All morphometric quantification was conducted with the investigator blind to genotype and treatment. Quantification of muscle endplate innervation Left and right gastrocnemius muscles from WT or adenoviral construct (GFP, human MyoD or human myogenin)-injected G93A mice were dissected and fixed in 4% PFA for 20 min on ice. Following incubation in 30% sucrose for 2 h, muscle was put in OCT and frozen using isopentane on dry ice. Frozen samples were stored at −80 °C until sectioned. Muscle samples were sectioned exhaustively on a cryostat at 40 μm thickness, mounted on to Super Frost slides (Fisher Scientific) and allowed to dry at RT for 10 min. Mounted sections were stored at −20 °C if short-term and at −80 °C if long-term. Every fourth section through the whole muscle was fluorescence-labelled for α-bungarotoxin, synaptophysin and neurofilament. Each muscle section was delineated using a stereology workstation, consisting of a Zeiss Imager M2 light microscope and a EC Plan Neofluar objective × 2.5 (numerical aperture (NA), 0.075) and a EC Plan Neofluar objective × 40 (NA, 0.75; Zeiss, Göttingen, Germany) to count. For counting, a motorized specimen stage for automatic sampling (MAX6000; Ludl Electronics, Hawthorne, NY), CCD colour video camera (CX9000; Microfire Digital CCD video camera) and stereology software (StereoInvestigator 9.0; MBF Bioscience, Williston, VT) were utilized. Total endplate number was determined from StereoInvestigator 9.0 using the physical fractionator probe with a grid size of 400 × 400 μm and counting frame of 100 × 100 μm. The percentage of innervated, intermediate and denervated endplates was determined as the total number of endplates divided by the number of innervated (overlapping synaptophysin and α-bungarotoxin staining), intermediate (no overlap but synaptophysin staining was adjacent to α-bungarotoxin) or denervated (no overlap and no apparent synaptophysin staining adjacent to α-bungarotoxin staining) endplates. Overall, the coefficient of error (CE) was <0.1. The investigator conducted the stereological analysis blind to genotype and treatment. Statistics Two-way ANOVA with Bonferroni post hoc test, one-way ANOVA, two-tailed unpaired t -test and Kaplan–Meier survival analysis were performed using Prism 4 for Macintosh (Prism v. 4.0, GraphPad Software Inc., San Diego, CA, USA). How to cite this article: Park, K.H.J. et al. Postnatal muscle modification by myogenic factors modulates neuropathology and survival in an ALS mouse model. Nat. Commun. 4:2906 doi: 10.1038/ncomms3906 (2013).